Identification of a subnuclear body involved in sequence-specific cytokine RNA processing Processing of interleukin RNAs must be tightly controlled during the immune response. Here we report that a subnuclear body called the interleukin-6 and -10 splicing activating compartment (InSAC) is a nuclear site of cytokine RNA production and stability. Tat-activating regulatory DNA-binding protein-43 (TDP-43) acts as an InSAC scaffold that selectively associates with IL-6 and IL-10 RNAs in a sequence-specific manner. TDP-43 also recruits key spliceosomal components from Cajal bodies. LPS induces posttranslational modifications of TDP-43; in particular, TDP-43 ubiquitination provides a driving force for InSAC formation. As a consequence, in vivo depletion of TDP-43 leads to a dramatic reduction in the RNA processing and the protein levels of IL-6 in serum. Collectively, our findings highlight the importance of TDP-43-mediated InSAC biogenesis in immune regulation. The mammalian nucleus is a complex organelle populated by many dynamic subcellular compartments in which numerous biological processes occur, including RNA transcription, splicing and degradation [1] , [2] . Several different types of nuclear bodies have been identified; however, the molecular mechanisms associated with most of these remain largely unknown [3] . The Cajal body (CB) is a nuclear compartment involved in the assembly of spliceosomal small-nuclear ribonucleoproteins (snRNPs) and telomere synthesis [4] , [5] , [6] , [7] . CBs are highly enriched in CB-specific small RNAs, which guide small nuclear RNA (U snRNA) modifications, and p80-coilin, which provides a structural scaffold through self-association [8] , [9] , [10] . Cytokines are proteins that act as signalling molecules to regulate immune responses and modulate cellular activities such as growth, survival and differentiation. In particular, interleukin (IL)-6 is a pluripotent cytokine that is involved in multiple pro- and anti-inflammatory processes [11] . In addition, IL-10 is an immune-regulatory cytokine critical for maintaining immune system balance through inhibiting the secretion of pro-inflammatory cytokines, preventing the production of Th1 cytokines (for example, IL-2 and interferon (IFN)-γ) and controlling the proliferation of B cells, T cells and macrophages [12] . Therefore, IL-6 and IL-10 messenger RNA production must be carefully regulated at practically all levels, as misregulated cytokine expression is known to be related to various autoimmune diseases, tumour growth and obesity [11] , [13] , [14] . However, a key regulatory molecular complex associated with cytokine RNA processing has not been identified. Tat-activating regulatory DNA-binding protein-43 (TDP-43 or Tardbp) was first identified as a DNA-binding protein with a putative role in HIV transcription [15] . TDP-43 is a highly conserved nucleic acid-binding protein that contains a characteristic amino-terminal domain, two RNA recognition motifs and a glycine-rich carboxy-terminal domain. It is involved in early embryogenesis, fat storage and in multiple events of RNA metabolism [16] , [17] , [18] , [19] , [20] , [21] . TDP-43 resides predominantly in the nucleus, but it localizes to the cytoplasm and aggregates as inclusion bodies in patients afflicted with amyotrophic lateral sclerosis (ALS) or frontotemporal lobar degeneration (FTLD) with ubiquitin-positive inclusions [22] , [23] . In pathological conditions, TDP-43 is also hyperphosphorylated and cleaved to generate C-terminal fragments of ~25 kDa [22] . In addition, TDP-43 overexpression causes neurotoxic effects, such as mitochondria aggregation, motor deficit, myelin degeneration or neuroinflammation [24] , [25] , [26] . However, the molecular function of TDP-43 in cytokine RNA processing occurring during the immune response remains to be elucidated. Here we describe the TDP-43-mediated interleukin-6 and -10 splicing activating compartment (InSAC) as the essential nuclear site of IL-6 or IL-10 mRNA production and stability. TDP-43 acts as a scaffold in the InSAC that interacts with IL-6 or IL-10 RNA, and recruits snRNAs and snRNPs from CBs. These functions facilitate pre-mRNA processing and prevent its degradation. Furthermore, lipopolysaccharide (LPS)-induced ubiquitination of TDP-43 provides a driving force in InSAC formation. Therefore, we propose that the biogenesis of InSAC functions as a specific cytokine-splicing compartment that is critical for efficient RNA production during the activation and modulation of the immune response. Identification of a novel TDP-43-enriched subnuclear body To study the role(s) of TDP-43 in the immune response, we first examined its subcellular localization in RAW 264.7 macrophages following stimulation with 80 ng ml −1 LPS for 2 or 6 h, which promotes robust cytokine production to induce innate and adaptive immunity [27] . As TDP-43 is known to reside primarily in the nucleoplasm, it was surprising to discover that stably expressed green fluorescence protein (GFP)-tagged TDP-43 was distributed sparsely throughout the nucleoplasm, but dramatically enriched within the spherical subnuclear foci in LPS-stimulated RAW macrophages ( Fig. 1a , arrowheads). We also noted that TDP-43-enriched subnuclear foci increased in size in a time-dependent manner. Approximately 45% of these cells exhibited one or two TDP-43-enriched foci in the nucleus, resembling CBs. To test whether LPS affects TDP-43 expression levels, we examined endogenous expression levels of TDP-43 in LPS-stimulated RAW macrophages, but no differences in TDP-43 expression were observed ( Fig. 1b ). Endogenous TDP-43 was also enriched within subnuclear foci following LPS stimulation, with smaller amounts distributed throughout the nucleoplasm ( Fig. 1c (a–f) ). To confirm the de novo formation of TDP-43 foci in response to LPS in primary cells, we examined endogenous TDP-43 in LPS-stimulated bone marrow-derived dendritic cells (BMDCs) ( Fig. 1c (g–l) ). Our data also showed the presence of TDP-43-enriched subnuclear foci following LPS exposure in primary BMDCs. 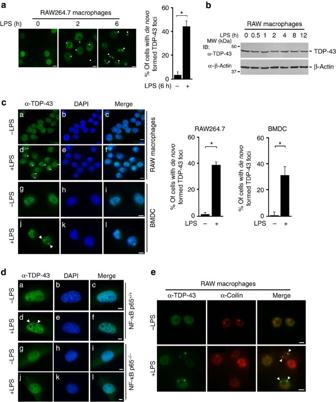Figure 1: LPS can induce thede novoformation of TDP-43 foci. (a) Immunofluorescence microscopy assay (IFA) of stable GFP-TDP-43-expressing RAW 264.7 macrophages following exposure to LPS (80 ng ml−1) for 2 or 6 h. Quantitative analysis ofde novoTDP-43 foci formation. Values represent the average (n=100–120 cells) of three independent experiments. Arrowheads indicate TDP-43-enriched subnuclear foci. Scale bars, 5 μm. *P<0.01 (two-tailed Student’st-test). (b) RAW macrophages were stimulated with LPS (80 ng ml−1) for the indicated times. Cell lysates were immunoblotted with anti-TDP-43 or anti-β-actin antibody. (c) LPS stimulation (80 ng ml−1) for 6 h leads to the enrichment of endogenous TDP-43 in subnuclear sites of RAW macrophages and primary BMDCs. Anti-TDP-43 primary antibody was used, along with Alexa 488-conjugated secondary antibody and 4′,6-diamidino-2-phenylindole (DAPI). Scale bars, 5 μm. Quantitative analysis ofde novoTDP-43-enriched foci formation. Values represent the average (n=100 cells) of three independent experiments. *P<0.05 (Student’st-test). (d) TDP-43 foci do not appear in NF-κB-deficient MEFs in the presence of LPS (80 ng ml−1). Endogenous TDP-43 was observed by anti-TDP-43 antibody. Scale bars, 5 μm. (e) Macrophages containing TDP-43-enriched nuclear foci display disrupted CB formation. RAW macrophages were exposed to LPS (80 ng ml−1) for 6 h, stained with anti-TDP-43 and anti-coilin antibody, and examined by IFA assay. Arrowheads indicate TDP-43-enriched foci. Scale bars, 5 μm. Data are representative of at least three independent experiments (mean±s.d. inaandc). Figure 1: LPS can induce the de novo formation of TDP-43 foci. ( a ) Immunofluorescence microscopy assay (IFA) of stable GFP-TDP-43-expressing RAW 264.7 macrophages following exposure to LPS (80 ng ml −1 ) for 2 or 6 h. Quantitative analysis of de novo TDP-43 foci formation. Values represent the average ( n =100–120 cells) of three independent experiments. Arrowheads indicate TDP-43-enriched subnuclear foci. Scale bars, 5 μm. * P <0.01 (two-tailed Student’s t -test). ( b ) RAW macrophages were stimulated with LPS (80 ng ml −1 ) for the indicated times. Cell lysates were immunoblotted with anti-TDP-43 or anti-β-actin antibody. ( c ) LPS stimulation (80 ng ml −1 ) for 6 h leads to the enrichment of endogenous TDP-43 in subnuclear sites of RAW macrophages and primary BMDCs. Anti-TDP-43 primary antibody was used, along with Alexa 488-conjugated secondary antibody and 4′,6-diamidino-2-phenylindole (DAPI). Scale bars, 5 μm. Quantitative analysis of de novo TDP-43-enriched foci formation. Values represent the average ( n =100 cells) of three independent experiments. * P <0.05 (Student’s t -test). ( d ) TDP-43 foci do not appear in NF-κB-deficient MEFs in the presence of LPS (80 ng ml −1 ). Endogenous TDP-43 was observed by anti-TDP-43 antibody. Scale bars, 5 μm. ( e ) Macrophages containing TDP-43-enriched nuclear foci display disrupted CB formation. RAW macrophages were exposed to LPS (80 ng ml −1 ) for 6 h, stained with anti-TDP-43 and anti-coilin antibody, and examined by IFA assay. Arrowheads indicate TDP-43-enriched foci. Scale bars, 5 μm. Data are representative of at least three independent experiments (mean±s.d. in a and c ). Full size image Next, we examined whether there are cell type-specific aspects to the de novo formation of TDP-43 foci. For those experiments, we assessed the formation of TDP-43 in activated CD4 + T cells, which are major producers of IFN-γ, and N2A (murine neuroblastoma) cells, which can naturally produce a large amount of IL-6 (ref. 28 ). Interestingly, TDP-43 foci were readily detectable in N2A cells even without LPS stimulation, but not in CD4 + effector T cells ( Supplementary Fig. 1a ). These results led us to hypothesize that the formation of TDP-43 foci is dependent on the specific cytokine RNA species produced in the cells rather than on the cell type or signal. To further investigate this possibility, we examined whether TDP-43 foci can form in nuclear factor-κB (NF-κB)-deficient mouse embryonic fibroblast (MEF) cells, which do not produce proinflammatory cytokines such as IL-6 or tumour necrosis factor (TNF)-α, in the presence of LPS ( Fig. 1d and Supplementary Fig. 1b ). We observed a lack of TDP-43 foci formation in NF-κB-deficient MEFs ( Fig. 1d (j) ). In addition, IL-6 was highly produced by N2A cells even in the absence of LPS, but not secreted by CD4 + T cells ( Supplementary Fig. 1c ), further supporting our hypothesis that the formation of TDP-43 foci is linked to the production of proinflammatory cytokines. As the de novo formation of TDP-43 subnuclear foci and that of CBs in LPS-stimulated cells are indistinguishable in size, shape and density, we next investigated whether the localization of LPS-mediated subnuclear TDP-43 foci formation overlapped with expression of the CB-specific marker p80-coilin. In LPS-stimulated macrophages, TDP-43 localization did not overlap with coilin ( Fig. 1e ). Surprisingly, CBs were disrupted in macrophages where TDP-43 was strongly enriched in subnuclear bodies ( Fig. 1e , see white arrowheads). We also examined TDP-43 localization with respect to other subnuclear compartments, such as nucleoli and promyelocytic leukemia bodies ( Supplementary Fig. 1d ). However, none of these overlapped with TDP-43 foci, suggesting that the TDP-43-enriched body represents a novel subnuclear compartment that forms de novo in response to LPS stimulation. TDP-43 is required for IL-6 RNA processing and stability To explore the function(s) of TDP-43 in innate immunity against microbial infection, we investigated the ability of TDP-43 to induce proinflammatory cytokine production in response to LPS stimulation. TDP-43 was depleted in primary BMDCs or bone marrow-derived macrophages (BMDMs) using TDP-43-specific small interfering RNA (siRNA). Notably, this depletion impaired the LPS-induced production of IL-6 but not that of TNF-α ( Fig. 2a ). Likewise, LPS-stimulated RAW macrophages stably expressing TDP-43-specific short hairpin RNA (shRNA) exhibited dramatically reduced production of IL-6 but not TNF-α ( Supplementary Fig. 2a ). We also observed a significant decrease of TDP-43 foci formation in TDP-43-depleted RAW macrophages ( Supplementary Fig. 2b ). As TDP-43 is involved in RNA metabolism, we next examined the effect of TDP-43 depletion on cytokine mRNA production by reverse transcription–PCR (RT–PCR) with the indicated primer pairs ( Supplementary Fig. 2c ). The quantity of IL-6 mRNA elicited by LPS stimulation was reduced markedly in TDP-43-depleted BMDMs; in contrast, TNF-α mRNA levels were unaffected ( Fig. 2b , indicated by arrowheads). Moreover, TDP-43 depletion led to the accumulation of unspliced IL-6 pre-mRNA and significant impairment of its processing ( Fig. 2b , arrows). We quantified the band intensity of their pre-mRNA or mRNA and showed that the sum of band intensity of mRNA and pre-mRNA from control cells was similar to that from TDP-43-depleted cells. Densitometric analysis also showed the accumulated amount of IL-6 pre-mRNA in TDP-43-depleted cells ( Fig. 2b , right graphs), suggesting that TDP-43 is a critical nuclear factor involved in IL-6 pre-mRNA processing. Quantitative RT–PCR (qRT–PCR) confirmed that TDP-43-depleted BMDMs showed a significant and reproducible reduction in IL-6 mRNA, but not that of TNF-α ( Fig. 2c ). We noted similar effects on IL-6 mRNA splicing in TDP-43-depleted RAW macrophages ( Supplementary Fig. 2d ). 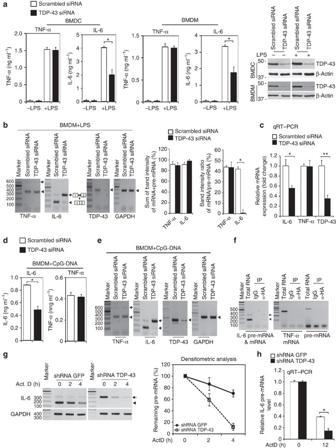Figure 2: TDP-43 is essential for IL-6 pre-mRNA processing and stability. (a,d) BMDMs or BMDCs were transfected with scrambled or TDP-43-specific siRNA. After treatment with LPS (80 ng ml−1) (a) or CpG-DNA (1 μM) (d) for 6 h, ELISA assay was carried out. *P<0.01 (Student’st-test). (b,e) RT–PCR for the exon–exon junction of the indicated cytokines was performed from LPS- or CpG-DNA-stimulated BMDMs expressing scrambled or TDP-43 siRNA. RT–PCR with the indicated primers (P1, P4, P6 or P7) for IL-6, TNF-α, TDP-43 and GAPDH yielded products of 167, 340, 405 and 376 bp, respectively, as predicted. P (No.) refers to the primer number for the indicated genes (Supplementary Fig. 2candSupplementary Table 1). Arrowheads and arrows indicate mRNA and pre-mRNA, respectively. Quantification of the band intensity of mRNA and pre-mRNA of IL-6 or TNF-α (right graphs). *P<0.005 (Student’st-test). (c) qRT–PCR using primer pairs (P2, P4 or P6) confirmed statistically significant reduction in IL-6 mRNA levels in TDP-43-depleted primary macrophages. All qRT–PCR data were normalized to GAPDH mRNA expression.*P<0.005 and **P<0.001 (Student’st-test). (f) TDP-43 binds IL-6 pre-mRNA or mRNA, but not TNF-α pre-mRNA or mRNA. RAW macrophages expressing HA-TDP-43 were exposed to LPS (80 ng ml−1) for 6 h. Lysates were immunoprecipitated with either anti-HA or anti-isotype antibody, and then subjected to RIP assay using the indicated primer pairs. RT–PCR with primer pairs (P1, P4 or P5) for IL-6 pre-mRNA/mRNA, TNF-α mRNA or TNF-α pre-mRNA, respectively, yielded 337/167, 340 or 448-bp products, as predicted for the RIP assay. Arrow and arrowheads indicate direct TDP-43 interaction with IL-6 pre-mRNA and mRNA. (g) The effect of TDP-43 depletion on pre-mRNA stability in LPS-stimulated macrophages was assessed by RT–PCR analysis of IL-6 pre-mRNA levels using primer pair P1. RNA was isolated at different time points after Act.D (5 μg ml−1) treatment. Densitometric analysis of the bands obtained in control or TDP-43-depleted cells. (h) qRT–PCR revealed the presence of unstable IL-6 pre-mRNA in TDP-43-depleted RAW macrophages.*P<0.01 (Student’st-test). Data are representative of more than three independent experiments (mean±s.d. ina,b,dandg; mean±s.e.m. incandh). Figure 2: TDP-43 is essential for IL-6 pre-mRNA processing and stability. ( a , d ) BMDMs or BMDCs were transfected with scrambled or TDP-43-specific siRNA. After treatment with LPS (80 ng ml −1 ) ( a ) or CpG-DNA (1 μM) ( d ) for 6 h, ELISA assay was carried out. * P <0.01 (Student’s t -test). ( b , e ) RT–PCR for the exon–exon junction of the indicated cytokines was performed from LPS- or CpG-DNA-stimulated BMDMs expressing scrambled or TDP-43 siRNA. RT–PCR with the indicated primers (P1, P4, P6 or P7) for IL-6, TNF-α, TDP-43 and GAPDH yielded products of 167, 340, 405 and 376 bp, respectively, as predicted. P (No.) refers to the primer number for the indicated genes ( Supplementary Fig. 2c and Supplementary Table 1 ). Arrowheads and arrows indicate mRNA and pre-mRNA, respectively. Quantification of the band intensity of mRNA and pre-mRNA of IL-6 or TNF-α (right graphs). * P <0.005 (Student’s t -test). ( c ) qRT–PCR using primer pairs (P2, P4 or P6) confirmed statistically significant reduction in IL-6 mRNA levels in TDP-43-depleted primary macrophages. All qRT–PCR data were normalized to GAPDH mRNA expression. *P <0.005 and ** P <0.001 (Student’s t -test). ( f ) TDP-43 binds IL-6 pre-mRNA or mRNA, but not TNF-α pre-mRNA or mRNA. RAW macrophages expressing HA-TDP-43 were exposed to LPS (80 ng ml −1 ) for 6 h. Lysates were immunoprecipitated with either anti-HA or anti-isotype antibody, and then subjected to RIP assay using the indicated primer pairs. RT–PCR with primer pairs (P1, P4 or P5) for IL-6 pre-mRNA/mRNA, TNF-α mRNA or TNF-α pre-mRNA, respectively, yielded 337/167, 340 or 448-bp products, as predicted for the RIP assay. Arrow and arrowheads indicate direct TDP-43 interaction with IL-6 pre-mRNA and mRNA. ( g ) The effect of TDP-43 depletion on pre-mRNA stability in LPS-stimulated macrophages was assessed by RT–PCR analysis of IL-6 pre-mRNA levels using primer pair P1. RNA was isolated at different time points after Act.D (5 μg ml −1 ) treatment. Densitometric analysis of the bands obtained in control or TDP-43-depleted cells. ( h ) qRT–PCR revealed the presence of unstable IL-6 pre-mRNA in TDP-43-depleted RAW macrophages. *P <0.01 (Student’s t -test). Data are representative of more than three independent experiments (mean±s.d. in a , b , d and g ; mean±s.e.m. in c and h ). Full size image To explore whether Toll-like receptor (TLR)-agonist specificity is involved in TDP-43-mediated IL-6 pre-mRNA processing, we measured cytokine production in purified BMDMs exposed to CpG-DNA, which activates the TLR9 signalling cascade. In TDP-43-depleted BMDMs, production of IL-6, but not TNF-α, was attenuated in response to CpG-DNA in a manner similar to LPS ( Fig. 2d ). Furthermore, induction of IL-6 RNA processing by CpG-DNA was severely impaired by loss of TDP-43 expression, while TNF-α RNA splicing remained unaffected ( Fig. 2e ). Based on these data, we hypothesized that TDP-43 must interact with IL-6 pre-mRNA to play a role in its RNA processing. To address this, we conducted IL-6 RNA pull-down analysis using LPS-stimulated RAW macrophages. Although the total amount of IL-6 pre-mRNA was much less than that of mRNA, RT–PCR clearly showed that TDP-43 strongly interacted with IL-6 pre-mRNA and only bound a very small amount of IL-6 mRNA ( Fig. 2f ). In contrast, TDP-43 did not interact with TNF-α mRNA or its pre-mRNA. These results also suggest another possible role for TDP-43 in regulating IL-6 pre-mRNA or mRNA stability. Unfortunately, it was not possible to examine IL-6 mRNA stability in TDP-43-depleted macrophages, because the impairment in pre-mRNA splicing reduced the level of IL-6 mRNA to an undetectable level. However, the half-life of IL-6 pre-mRNA in TDP-43-depleted macrophages was much shorter than in control macrophages ( Fig. 2g,h ). Therefore, we conclude that TDP-43 is essential for IL-6 pre-mRNA processing and stability. TDP-43 binds IL-6 or IL-10 RNA Previous studies have shown that TDP-43 preferentially binds pre-mRNA [21] . As TDP-43 plays a role in processing IL-6 but not TNF-α RNA ( Fig. 2 ), it is possible that TDP-43 may bind IL-6 RNA in a sequence-dependent manner during processing. As previous reports demonstrated TDP-43 binding to long clusters of UG-rich sites in the brain [20] , [21] , we first compared the intronic sequences of IL-6 and TNF-α RNA, to examine whether IL-6 contains UG-rich sequences within its introns. We found that IL-6 contained several UG-rich sequences within introns 1, 2 and 4; however, we also easily found UG-rich sequences within the intronic regions of TNF-α, indicating that TDP-43 may not use these sites to bind IL-6 RNA. To identify the putative TDP-43-binding region(s) in IL-6 RNA, we designed primer pairs corresponding to each intron of IL-6 RNA for an RNA immunoprecipitation (RIP) assay ( Fig. 3a ). As the long strands of IL-6 pre-mRNA are relatively unstable in the absence of TDP-43 binding to introns, unbound RNA may be easily cleaved and susceptible to degradation during the RIP assay. We detected an interaction between TDP-43 and IL-6 introns 1 or 2, but not introns 3 or 4 ( Fig. 3b ). To further identify specific sequence(s) within IL-6 introns 1 or 2 targeted by TDP-43, we applied RNA secondary structure prediction programmes (CentroidFold, www.ncRNA.org ). Surprisingly, this analysis revealed that intron 2 of mouse IL-6 contains a predicted stem-loop structure consisting of GC-rich palindromic repeats and a short spacer consisting of ‘GCACU’ ( Fig. 3c and Supplementary Fig. 3 ). Introns 2 and 3 of TNF-α, as well as introns 3 and 4 of IL-6, each contain a similar sequence; however, it was distinct from that of IL-6 intron 2, as they contain short GC- or AT-rich palindromic sequences and a large loop ( Supplementary Fig. 3 ). Next, we analysed all the introns present in RNAs for other cytokines, including TNF-α, IL-1β, IL-4, IL-8, IL-10, IL-12, IFN-α, IFN-β and IFN-γ, to determine whether they contain this predicted sequence. Notably, intron 1 of mouse IL-10 contained GC-rich palindromic repeats and a short spacer including ‘ACU’, similar to mouse IL-6 ( Fig. 3c and Supplementary Figs 3 and 4 ). However, we did not observe any conserved sequences among the intronic sequences of TNF-α, IL-1β, IL-4, IL-8, IL-12, IFN-α, IFN-β or IFN-γ ( Supplementary Fig. 3 ). 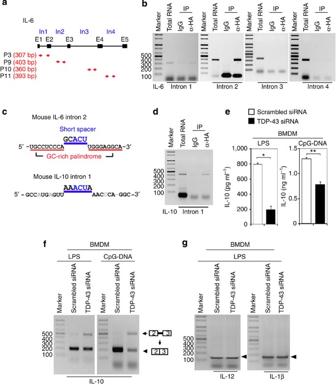Figure 3: TDP-43 interacts specifically with IL-6 and IL-10 RNAs. (a) Schematic representation of various primer pairs corresponding to each intron of IL-6 RNA and the predicted size of RT–PCR products for the RIP assay. Red arrows indicate the primer annealing sites and the predicted sizes of the RT–PCR product. (b) Intron 2 of IL-6 RNA is a putative binding region of TDP-43. RAW macrophages expressing HA-TDP-43 were exposed to LPS (80 ng ml−1) for 6 h. Lysates were immunoprecipitated with anti-HA or anti-isotype antibody and then subjected to the RIP assay using the indicated primers ina. (c) Sequences of IL-6 and IL-10, containing a predicted binding sequence composed of GC-rich palindromic repeats and the conserved sequence motif ‘ACU’ in a short spacer region. (d) TDP-43 binds IL-10 intron 1 containing a specific binding sequence. RT–PCR of macrophages with primers (P12) against IL-10 intron 1 generated a 427-bp product as predicted. RAW macrophages were used for RIP assay. (e) After treatment with LPS (80 ng ml−1) or CpG-DNA (1 μM) into BMDMs for 6 h, ELISA assay was carried out to measure IL-10 levels in culture supernatants.*P<0.005 and**P<0.01 (Student’st-test). (f,g) Effect of TDP-43 depletion on IL-10, IL-12 or IL-1β RNA processing in LPS- or CpG-DNA-stimulated primary BMDMs was assessed by RT–PCR analysis with primer pairs (P13, P14 or P15, seeSupplementary Fig. 5a). RT–PCR with the indicated primer pairs for IL-10, IL-12 or IL-1β generated 191-, 144- or 163-bp products, respectively, as predicted (seeSupplementary Table 1). Data are from at least three independent experiments (mean±s.d. ine). Figure 3: TDP-43 interacts specifically with IL-6 and IL-10 RNAs. ( a ) Schematic representation of various primer pairs corresponding to each intron of IL-6 RNA and the predicted size of RT–PCR products for the RIP assay. Red arrows indicate the primer annealing sites and the predicted sizes of the RT–PCR product. ( b ) Intron 2 of IL-6 RNA is a putative binding region of TDP-43. RAW macrophages expressing HA-TDP-43 were exposed to LPS (80 ng ml −1 ) for 6 h. Lysates were immunoprecipitated with anti-HA or anti-isotype antibody and then subjected to the RIP assay using the indicated primers in a . ( c ) Sequences of IL-6 and IL-10, containing a predicted binding sequence composed of GC-rich palindromic repeats and the conserved sequence motif ‘ACU’ in a short spacer region. ( d ) TDP-43 binds IL-10 intron 1 containing a specific binding sequence. RT–PCR of macrophages with primers (P12) against IL-10 intron 1 generated a 427-bp product as predicted. RAW macrophages were used for RIP assay. ( e ) After treatment with LPS (80 ng ml −1 ) or CpG-DNA (1 μM) into BMDMs for 6 h, ELISA assay was carried out to measure IL-10 levels in culture supernatants. *P <0.005 and **P <0.01 (Student’s t -test). ( f , g ) Effect of TDP-43 depletion on IL-10, IL-12 or IL-1β RNA processing in LPS- or CpG-DNA-stimulated primary BMDMs was assessed by RT–PCR analysis with primer pairs (P13, P14 or P15, see Supplementary Fig. 5a ). RT–PCR with the indicated primer pairs for IL-10, IL-12 or IL-1β generated 191-, 144- or 163-bp products, respectively, as predicted (see Supplementary Table 1 ). Data are from at least three independent experiments (mean±s.d. in e ). Full size image If this predicted stem-loop sequence is required for TDP-43 binding, then TDP-43 should interact physically with IL-10 intron 1. To address this hypothesis, we performed IL-10 pre-mRNA pull-down assays in LPS-stimulated macrophages. Indeed, TDP-43 interacted with IL-10 pre-mRNA ( Fig. 3d ). Our data also demonstrate that this factor plays a role in IL-10 production and RNA processing, because TDP-43-depleted BMDMs exhibited lower IL-10 secretion in response to LPS stimulation ( Fig. 3e ), as well as accumulation of unspliced IL-10 pre-mRNA and a significant defect in its processing in primary cells following LPS or CpG-DNA treatment ( Fig. 3f ). To confirm these results, we assessed IL-10 production in LPS-stimulated RAW macrophages stably expressing TDP-43 shRNA. As expected, both IL-10 production and RNA processing were significantly reduced in TDP-43-depleted macrophages ( Supplementary Fig. 5b,c ). However, TDP-43 knockdown did not affect the processing of IL-12 or IL-1β RNA, which do not contain a specific sequence, as the amount of mRNA was similar in BMDMs expressing TDP-43 siRNA and scrambled siRNA ( Fig. 3g ). Taken together, we conclude that TDP-43 can recognize a specific sequence that contains a GC-rich palindromic repeat with the conserved ‘ACU’ sequence motif in a short spacer that forms a putative stem-loop. TDP-43 promotes IL-6 and IL-10 RNA processing If TDP-43 binds IL-6 and IL-10 RNAs in a sequence-specific manner, then synthetic RNA containing these features should interact with TDP-43 directly in vitro . We examined the interaction of TDP-43 with a biotinylated synthetic RNA sequence encompassing nucleotides 521–543 of mouse IL-6 intron 2, which consists of a GC-rich palindromic sequence and the conserved sequence motif ‘ACU’ in a short spacer ( Supplementary Fig. 4 ). A mutated synthetic IL-6 RNA composed of a sequence designed to disrupt the palindromic sequences and conserved sequence motif (mutCA+GUUUCUU) in a spacer was also examined. Indeed, TDP-43 interacted with the synthetic wild-type RNA containing the intact conserved sequences, but not with the mutated RNA ( Fig. 4a , right panels). To confirm the specificity of this interaction, we further investigated the interaction of TDP-43 with mutated RNAs in which ‘AC’ was substituted with ‘GU’ in the conserved sequence motif (ACU) of a short spacer region (mutGU), or ‘GGG’ with ‘UUU’ in a GC-rich palindromic repeat (mutUUU) ( Fig. 4b , upper schematic sequences). Unlike wild-type IL-6 RNA, TDP-43 did not bind to either mutGU or mutUUU ( Fig. 4b ). 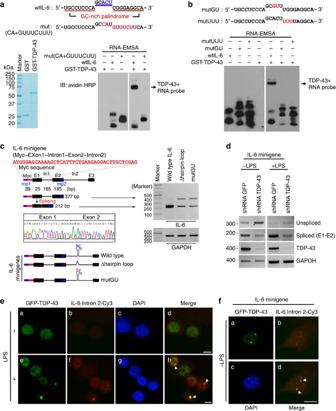Figure 4: TDP-43 promotes IL-6 RNA processing in a stem-loop-dependent manner. (a) Top, schematic representation of the sequences of wild-type IL-6 intron 2 and mutant IL-6 RNAs. mutCA+GUUUCUU, a mutated synthetic IL-6 RNA composed of a sequence designed to disrupt the palindromic region and conserved sequence motif in a short spacer. Red letters indicate mutated sequences. Bottom, a predicted stem-loop sequence in IL-6 RNA is required for TDP-43 interactionin vitro. Purified GST-fused TDP-43 incubated with either synthetic wild-type or mutant IL-6 RNA (mutCA+GUUUCUU). Both synthetic RNAs were conjugated to biotin, allowing detection of the TDP-43 interaction with synthetic RNAs. (b) Top, schematic representation of the sequences of mutGU; a substitution of ‘AC’ to ‘GU’ in the conserved sequence motif ‘ACU’ of the short-spacer region, mutUUU; point mutation of ‘GGG’ to ‘UUU’ in a GC-rich palindromic sequence. Red letters indicate mutated sequences. Bottom, purified GST-fused TDP-43 incubated with either synthetic wild-type IL-6 RNA or mutant RNAs (mutGU and mutUUU). TDP-43-RNA binding was performed using the RNA electrophoretic mobility shift assay (RNA EMSA) assay. (c) Schematic representation of the IL-6 minigene containing exons 1, 2 and 3 along with introns 1 and 2. RT–PCR with a forward primer (mp1) corresponding to the 5′-Myc tag and a reverse primer (mp2) for exon 2 generated 212-bp (Myc and exons 1 and 2) or 377-bp (Myc, exons 1 and 2 plus intron 1) products, as predicted. (d) RT–PCR of TDP-43-depleted LPS-stimulated and unstimulated macrophages expressing the wild-type IL-6 minigene. (e) TDP-43 foci contain IL-6 pre-mRNA in LPS-stimulated RAW macrophages. RNA-FISH showing co-localization of TDP-43-enriched foci with an IL-6 intron 2-specific antisense oligo probe conjugated to Cy3. Scale bars, 5 μm. (f) TDP-43-mediated subnuclear foci form in RAW macrophages expressing the IL-6 minigene even in the absence of LPS-stimulation. Scale bars, 5 μm. Data are representative of three experiments (c–f), or are from four independent experiments (a,b). Figure 4: TDP-43 promotes IL-6 RNA processing in a stem-loop-dependent manner. ( a ) Top, schematic representation of the sequences of wild-type IL-6 intron 2 and mutant IL-6 RNAs. mutCA+GUUUCUU, a mutated synthetic IL-6 RNA composed of a sequence designed to disrupt the palindromic region and conserved sequence motif in a short spacer. Red letters indicate mutated sequences. Bottom, a predicted stem-loop sequence in IL-6 RNA is required for TDP-43 interaction in vitro . Purified GST-fused TDP-43 incubated with either synthetic wild-type or mutant IL-6 RNA (mutCA+GUUUCUU). Both synthetic RNAs were conjugated to biotin, allowing detection of the TDP-43 interaction with synthetic RNAs. ( b ) Top, schematic representation of the sequences of mutGU; a substitution of ‘AC’ to ‘GU’ in the conserved sequence motif ‘ACU’ of the short-spacer region, mutUUU; point mutation of ‘GGG’ to ‘UUU’ in a GC-rich palindromic sequence. Red letters indicate mutated sequences. Bottom, purified GST-fused TDP-43 incubated with either synthetic wild-type IL-6 RNA or mutant RNAs (mutGU and mutUUU). TDP-43-RNA binding was performed using the RNA electrophoretic mobility shift assay (RNA EMSA) assay. ( c ) Schematic representation of the IL-6 minigene containing exons 1, 2 and 3 along with introns 1 and 2. RT–PCR with a forward primer (mp1) corresponding to the 5′-Myc tag and a reverse primer (mp2) for exon 2 generated 212-bp (Myc and exons 1 and 2) or 377-bp (Myc, exons 1 and 2 plus intron 1) products, as predicted. ( d ) RT–PCR of TDP-43-depleted LPS-stimulated and unstimulated macrophages expressing the wild-type IL-6 minigene. ( e ) TDP-43 foci contain IL-6 pre-mRNA in LPS-stimulated RAW macrophages. RNA-FISH showing co-localization of TDP-43-enriched foci with an IL-6 intron 2-specific antisense oligo probe conjugated to Cy3. Scale bars, 5 μm. ( f ) TDP-43-mediated subnuclear foci form in RAW macrophages expressing the IL-6 minigene even in the absence of LPS-stimulation. Scale bars, 5 μm. Data are representative of three experiments ( c – f ), or are from four independent experiments ( a , b ). Full size image To define whether RNA sequence is critical for TDP-43-mediated IL-6 RNA processing, we constructed an N-terminal Myc-tagged IL-6 minigene that contains exons 1, 2 and 3 along with introns 1 and 2, or mutated IL-6 minigenes that either lack the entire putative stem-loop region or possess ‘GU’ instead of ‘AC’ in the spacer region ( Fig. 4c ). RT–PCR analysis with a forward primer (mp1) corresponding to the 5′-Myc tag and a reverse primer (mp2) for exon 2 produced a 212-bp product, as expected, from the IL-6 minigene composed of the region from exon 1 to exon 2, which represents a spliced form of the wild-type IL-6 minigene. Even in the absence of LPS, spliced products were clearly detected in wild-type IL-6 minigene-expressing macrophages; however, the spliced form of the mutant minigene was reduced ( Fig. 4c , right panel). Furthermore, we analysed IL-6 RNA processing in TDP-43-depleted macrophages expressing the wild-type IL-6 minigene ( Fig. 4d ). TDP-43 knockdown caused a reduction in the spliced form of the wild-type IL-6 minigene; however, splicing was normal in the absence of LPS. These findings suggest that a specific sequence in IL-6 pre-mRNA is critical for TDP-43 binding selectivity and RNA processing. Moreover, LPS does not seem to be necessary for mediating IL-6 RNA processing. If TDP-43-enriched foci are involved in IL-6 RNA processing, they should contain IL-6 pre-mRNA for processing. To examine this possibility, we simultaneously performed RNA-fluorescence in situ hybridization (RNA-FISH) and immunolocalization in macrophages. Dual labelling of IL-6 pre-mRNA with Cy3 and TDP-43 with GFP revealed that IL-6 pre-mRNA co-localized with TDP-43-positive foci in LPS-stimulated macrophages ( Fig. 4e , arrowheads). As TDP-43 foci were detected in N2A cells (even in the absence of LPS stimulation) but not in NF-κB-deficient cells ( Fig. 1d and Supplementary Fig. 1a ), and TDP-43-mediated RNA processing of the IL-6 minigene was independent of LPS-stimulation ( Fig. 4c,d ), we examined whether the formation of TDP-43 foci was indeed dependent on the presence of IL-6 RNA rather than LPS. We co-expressed GFP-TDP-43 and N-terminal Myc-tagged IL-6, IL-10 or TNF-α minigenes in macrophages and performed RNA-FISH with Cy3-IL-6, IL-10 or TNF-α pre-mRNA in the absence of LPS. Indeed, even without LPS stimulation, we observed the formation of TDP-43 foci containing IL-6 and IL-10 pre-mRNA, but not that of TNF-α ( Fig. 4f arrowheads, and Supplementary Fig. 5d arrowhead). Taken together, we conclude that the IL-6 and IL-10 RNA-binding selectivity of TDP-43 is due to the recognition of specific pre-mRNA sequence containing a GC-rich palindromic sequence and a conserved sequence motif within a short spacer region. This binding facilitates the processing of bound RNAs in TDP-43 foci. Based on this role, we named the TDP-43-enriched foci InSAC. InSAC recruits essential spliceosomal components To understand the detailed molecular mechanisms underlying InSAC formation in IL-6 pre-mRNA processing, we further examined whether the InSAC contains essential spliceosomal U snRNAs. RAW Macrophages were stimulated with LPS before protein extraction and immunoprecipitation with an anti-trimethylguanosine antibody that recognizes the 2, 2, 7-trimethylguanosine cap of snRNAs. Immunoprecipitates were probed in immunoblottings with an anti-TDP-43 or anti-coilin antibody. Remarkably, TDP-43 was found to be associated with snRNAs in LPS-treated macrophages. These cells also showed a disruption of the interaction between coilin and snRNAs ( Fig. 5a , upper and bottom panels, lanes 4 and 5). These results suggest that TDP-43 hijacks spliceosomal U snRNAs and recruits them to InSACs for the tight regulation of IL-6 and IL-10 pre-mRNA processing. 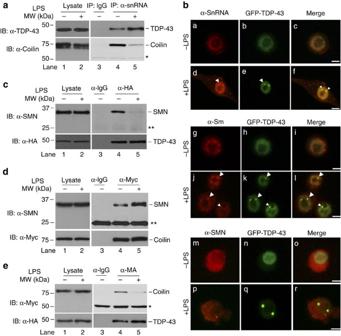Figure 5: TDP-43 is required for recruitment of critical spliceosomal components from CBs. (a) Effect of LPS stimulation on endogenous TDP-43 or coilin interaction with spliceosomal snRNAs. RAW macrophages were stimulated with LPS (80 ng ml−1) for 6 h and then lysed with 2% (v/v) NP-40. Supernatants were subjected to immunoprecipitation with anti-trimethylguanosine (snRNA) antibody before immunoblot analysis with anti-TDP-43 and then with anti-coilin antibody. (b) GFP-TDP-43 co-localizes with endogenous spliceosomal U snRNAs and Sm proteins, but not with SMN. RAW macrophages expressing GFP-TDP-43 were visualized by immunofluorescence microscopy using the indicated antibodies. White arrows indicate colocalization of TDP-43 with snRNAs or Sm proteins. Scale bars, 5 μm. (c,d) LPS stimulation reduced association of TDP-43 with SMN and increased binding of coilin with SMN. Cell extracts from LPS-stimulated RAW macrophages stably expressing HA-TDP-43 or coilin-Myc were immunoprecipitated with anti-HA or anti-Myc antibody, and then subjected to immunoblot analysis with anti-SMN antibody. The same blots were reprobed with anti-HA or anti-Myc antibody to verify the expression levels of TDP-43 or coilin. (e) The association of TDP-43 with coilin was disrupted by LPS stimulation. RAW macrophages stably expressing both HA-TDP-43 and coilin-Myc were incubated with LPS (80 ng ml−1), lysed with 2% NP-40 and then immunoprecipitated with anti-HA antibody before immunoblot analysis with anti-Myc antibody. *immunoglobulin heavy chains, **immunoglobulin light chains. Data are representative of at least three independent experiments. Figure 5: TDP-43 is required for recruitment of critical spliceosomal components from CBs. ( a ) Effect of LPS stimulation on endogenous TDP-43 or coilin interaction with spliceosomal snRNAs. RAW macrophages were stimulated with LPS (80 ng ml −1 ) for 6 h and then lysed with 2% (v/v) NP-40. Supernatants were subjected to immunoprecipitation with anti-trimethylguanosine (snRNA) antibody before immunoblot analysis with anti-TDP-43 and then with anti-coilin antibody. ( b ) GFP-TDP-43 co-localizes with endogenous spliceosomal U snRNAs and Sm proteins, but not with SMN. RAW macrophages expressing GFP-TDP-43 were visualized by immunofluorescence microscopy using the indicated antibodies. White arrows indicate colocalization of TDP-43 with snRNAs or Sm proteins. Scale bars, 5 μm. ( c , d ) LPS stimulation reduced association of TDP-43 with SMN and increased binding of coilin with SMN. Cell extracts from LPS-stimulated RAW macrophages stably expressing HA-TDP-43 or coilin-Myc were immunoprecipitated with anti-HA or anti-Myc antibody, and then subjected to immunoblot analysis with anti-SMN antibody. The same blots were reprobed with anti-HA or anti-Myc antibody to verify the expression levels of TDP-43 or coilin. ( e ) The association of TDP-43 with coilin was disrupted by LPS stimulation. RAW macrophages stably expressing both HA-TDP-43 and coilin-Myc were incubated with LPS (80 ng ml −1 ), lysed with 2% NP-40 and then immunoprecipitated with anti-HA antibody before immunoblot analysis with anti-Myc antibody. *immunoglobulin heavy chains, **immunoglobulin light chains. Data are representative of at least three independent experiments. Full size image To confirm the ability of TDP-43 to bind and recruit spliceosomal U snRNAs into InSACs, we examined the co-localization of TDP-43 with snRNAs in the InSACs by immunofluorescence microscopy. Endogenous U snRNAs were indeed co-localized with GFP-TDP-43 in LPS-stimulated macrophages and were therefore present in InSACs ( Fig. 5b (f) ). Moreover, components of spliceosomal snRNPs (SmB/B' and SmD1) were also found in the InSACs ( Fig. 5b (l) ). As the survival of motor neurons (SMN) complex is involved in snRNP assembly [29] , we next examined the co-localization of SMN with TDP-43. In macrophages, SMN tended to distribute within CBs as well as diffusely throughout the nucleoplasm and cytoplasm, and no differences in SMN localization were observed between LPS-stimulated versus unstimulated cells ( Fig. 5b (m,p) ). As a result, SMN was partially co-localized with TDP-43 throughout the nucleoplasm in unstimulated cells, but the distribution of SMN did not overlap with TDP-43-containing InSACs in LPS-stimulated macrophages ( Fig. 5b (r) ). We observed similar results from biochemical assays showing that TDP-43 bound to SMN in unstimulated cells, whereas LPS-treated macrophages showed a significant decrease in the association of these two proteins ( Fig. 5c , lanes 4 and 5). Surprisingly, the interaction between coilin and SMN increased with LPS stimulation ( Fig. 5d , lanes 4 and 5). In addition to observing a disruption in the formation of CBs, where TDP-43-mediated InSACs assemble de novo ( Fig. 1e ), the interaction between TDP-43 and coilin was also perturbed by LPS stimulation, as we had hypothesized ( Fig. 5e , lanes 4 and 5). Taken together, these results demonstrate that TDP-43 plays a role not only in competitively recruiting essential spliceosomal components to InSACs from CBs in response to LPS, but also in controlling the distribution of subnuclear compartments, including CBs, SMN complexes and InSACs. LPS induces posttranslational modifications of TDP-43 Previous studies have reported that cytoplasmic TDP-43 inclusions that form in neurons and astroglia of ALS and FTLD patients by a variety of factors are rich in ubiquitinated, oligomerized and hyperphosphorylated, and they are also cleaved to generate N- or C-terminal TDP-43 fragments [22] , [30] . We thus hypothesized that infectious stimulation may enhance the propensity of TDP-43 to undergo modification, which supports InSAC formation, and examined whether this protein undergoes any posttranslational modification in LPS-stimulated macrophages. The possibility of LPS-induced TDP-43 oligomerization was assessed in macrophages stably expressing GFP-TDP-43 and HA-TDP-43. Proteins from LPS-treated macrophages were immunoprecipitated with anti-HA antibody and then subjected to immunoblotting with anti-TDP-43 antibody. Notably, LPS facilitated TDP-43 oligomerization ( Fig. 6a , lane 3). Moreover, we found that TDP-43 in LPS-stimulated macrophages was cleaved into two different fragments ( Fig. 6b , arrowheads). To exclude the outcomes of nonspecific bands by LPS stimulation, we examined LPS-induced TDP-43 fragmentation in TDP-43-depleted cells. Based on the disappearance of the cleaved forms in TDP-43 knockdown cells, we conclude that these cleaved fragments were indeed generated from full-length TDP-43 in response to LPS. 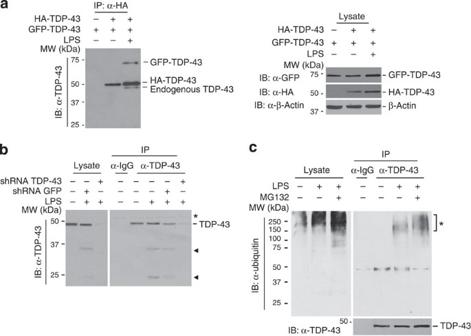Figure 6: LPS induces posttranslational modifications of TDP-43. (a) RAW macrophages stably expressing HA-TDP-43 and GFP-TDP-43 were stimulated with LPS (80 ng ml−1) for 6 h. Cell extracts were immunoprecipitated with anti-HA antibody and then subjected to immunoblot analysis with anti-TDP-43 antibody. TDP-43 expression was confirmed by immunoblot analysis using anti-HA, anti-GFP or anti-TDP-43 antibodies. (b) RAW macrophages were stimulated with LPS (80 ng ml−1), followed by immunoprecipitation with rat anti-TDP-43 antibody and probing with mouse anti-TDP-43 antibody. Asterisks and arrowheads indicate the immunoglobulin heavy chains and cleaved TDP-43, respectively. (c) RAW macrophages were stimulated with LPS (80 ng ml−1) and then treated with MG132 (10 μM). Cells were lysed with 2% NP-40, immunoprecipitated with anti-TDP-43 antibody and then analysed by immunoblotting with anti-ubiquitin antibody. Immunoprecipitated TDP-43 was confirmed by immunoblot analysis using anti-TDP-43 antibodies. Asterisk, ubiquitinated TDP-43. Data are representative of three independent experiments. Figure 6: LPS induces posttranslational modifications of TDP-43. ( a ) RAW macrophages stably expressing HA-TDP-43 and GFP-TDP-43 were stimulated with LPS (80 ng ml −1 ) for 6 h. Cell extracts were immunoprecipitated with anti-HA antibody and then subjected to immunoblot analysis with anti-TDP-43 antibody. TDP-43 expression was confirmed by immunoblot analysis using anti-HA, anti-GFP or anti-TDP-43 antibodies. ( b ) RAW macrophages were stimulated with LPS (80 ng ml −1 ), followed by immunoprecipitation with rat anti-TDP-43 antibody and probing with mouse anti-TDP-43 antibody. Asterisks and arrowheads indicate the immunoglobulin heavy chains and cleaved TDP-43, respectively. ( c ) RAW macrophages were stimulated with LPS (80 ng ml −1 ) and then treated with MG132 (10 μM). Cells were lysed with 2% NP-40, immunoprecipitated with anti-TDP-43 antibody and then analysed by immunoblotting with anti-ubiquitin antibody. Immunoprecipitated TDP-43 was confirmed by immunoblot analysis using anti-TDP-43 antibodies. Asterisk, ubiquitinated TDP-43. Data are representative of three independent experiments. Full size image Furthermore, immunoblot analysis with an anti-ubiquitin antibody revealed the presence of ubiquitinated endogenous TDP-43, which appeared as a large-molecular weight smear in the top panel (asterisk in Fig. 6c ). We also examined TDP-43 phosphorylation in macrophages exposed to LPS, but we did not observe such phosphorylation in response to LPS stimulation ( Supplementary Fig. 6a ). In addition, TDP-43 contains a putative sumoylation site (VKKD) within the amino acid region 135–138 ( Supplementary Fig. 6b ). To address the possibility of LPS-mediated TDP-43 sumoylation, we examined endogenous TDP-43 sumoylation in LPS-simulated cells. However, we did not observe any sumoylated TDP-43 in the absence or presence of LPS ( Supplementary Fig. 6c ). Based on these data taken together, we conclude that LPS promotes the oligomerization, fragmentation and ubiquitination of TDP-43, which may facilitate InSAC formation and nucleate the essential components of spliceosomal snRNPs and IL-6 or IL-10 RNA for efficient RNA processing. TDP-43 ubiquitination is essential for IL-6 RNA processing As many lines of evidence show that TDP-43 ubiquitination provides a strong driving force for the formation of intracellular inclusion bodies in ALS or FTLD, we focused on this modification and investigated whether the ubiquitination of TDP-43 is necessary for the formation of subnuclear InSAC and the processing of IL-6 RNA. In particular, as the ubiquitin-conjugating enzyme UBE2E3 regulates TDP-43 ubiquitination [31] , we generated macrophages stably expressing UBE2E3 shRNA and examined TDP-43 ubiquitination in LPS-stimulated macrophages. We clearly observed that UBE2E3 depletion reduced TDP-43 ubiquitination in the presence of LPS ( Fig. 7a ). Furthermore, in UBE2E3-depleted cells, the number of InSAC formed was significantly decreased, and the RNA processing and protein secretion of IL-6 were much lower than seen in control cells ( Fig. 7b–d ). Therefore, we conclude that TDP-43 ubiquitination is required for InSAC formation, thereby promoting IL-6 RNA processing. 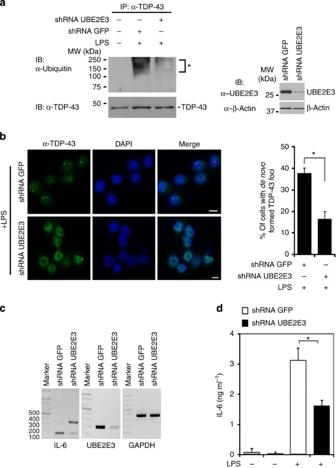Figure 7: TDP-43 ubiquitination is essential forde novoTDP-43 foci formation. (a) RAW macrophages stably expressing shRNA UBE2E3 or shRNA GFP were stimulated with LPS (80 ng ml−1) for 6 h. Lysate were immunoprecipitated with anti-TDP-43 antibody and then analysed by immunoblotting with anti-ubiquitin antibody. Immunoprecipitated TDP-43 was confirmed by immunoblot analysis using anti-TDP-43 antibodies. Asterisk, ubiquitinated TDP-43. The efficiency of UBE2E3 depletion was confirmed by immunoblot analysis anti-UBE2E3 or anti-β-actin antibody. (b) RAW macrophages stably expressing shRNA UBE2E3 or shRNA GFP were stimulated with LPS (80 ng ml−1) and stained with anti-TDP-43 and DAPI. Scale bars, 5 μm. Quantitative analysis ofde novoTDP-43-enriched foci formation. Values represent the average (n=150 cells) of three independent experiments.*P<0.01 (Student’st-test). (c) RAW macrophages stably expressing shRNA UBE2E3 or shRNA GFP were stimulated with LPS (80 ng ml−1) for 6 h. RT–PCR using primer pairs (P1) confirmed the statistically significant reduction in IL-6 mRNA levels in UBE2E3-depleted macrophages. The efficiency of UBE2E3 knockdown was confirmed by RT–PCR analysis. (d) ELISA was performed to measure IL-6 levels in culture supernatants from RAW macrophages expressing shRNA GFP or shRNA UBE2E3. ELISA confirmed the statistically significant decrease in IL-6 secretion levels in UBE2E3-depleted RAW macrophages.*P<0.001 (Student’st-test). Data are representative of three independent experiments (mean±s.d. inbandd). Figure 7: TDP-43 ubiquitination is essential for de novo TDP-43 foci formation. ( a ) RAW macrophages stably expressing shRNA UBE2E3 or shRNA GFP were stimulated with LPS (80 ng ml −1 ) for 6 h. Lysate were immunoprecipitated with anti-TDP-43 antibody and then analysed by immunoblotting with anti-ubiquitin antibody. Immunoprecipitated TDP-43 was confirmed by immunoblot analysis using anti-TDP-43 antibodies. Asterisk, ubiquitinated TDP-43. The efficiency of UBE2E3 depletion was confirmed by immunoblot analysis anti-UBE2E3 or anti-β-actin antibody. ( b ) RAW macrophages stably expressing shRNA UBE2E3 or shRNA GFP were stimulated with LPS (80 ng ml −1 ) and stained with anti-TDP-43 and DAPI. Scale bars, 5 μm. Quantitative analysis of de novo TDP-43-enriched foci formation. Values represent the average ( n =150 cells) of three independent experiments. *P <0.01 (Student’s t -test). ( c ) RAW macrophages stably expressing shRNA UBE2E3 or shRNA GFP were stimulated with LPS (80 ng ml −1 ) for 6 h. RT–PCR using primer pairs (P1) confirmed the statistically significant reduction in IL-6 mRNA levels in UBE2E3-depleted macrophages. The efficiency of UBE2E3 knockdown was confirmed by RT–PCR analysis. ( d ) ELISA was performed to measure IL-6 levels in culture supernatants from RAW macrophages expressing shRNA GFP or shRNA UBE2E3. ELISA confirmed the statistically significant decrease in IL-6 secretion levels in UBE2E3-depleted RAW macrophages. *P <0.001 (Student’s t -test). Data are representative of three independent experiments (mean±s.d. in b and d ). Full size image Effect of in vivo TDP-43 depletion on cytokine production To test the physiological effect of TDP-43 in cytokine RNA processing, we assessed IL-6 and TNF-α mRNA levels in live mice depleted of TDP-43 and injected with LPS to induce cytokine RNA production ( Fig. 8a ). In vivo delivery of target siRNA is a well-established system that allowed us to deplete TDP-43 systemically in live mice in vivo , especially in the spleen. Indeed, TDP-43 was significantly depleted in the splenic macrophages ( Fig. 8b,c ). Importantly, qRT–PCR demonstrated that TDP-43-depleted mice showed reduced IL-6 mRNA production. In contrast, we did not observe a significant difference in TNF-α RNA production on TDP-43 depletion ( Fig. 8c ). In addition, IL-6 RNA processing was also markedly impaired by in vivo TDP-43 depletion ( Fig. 8d ). Furthermore, we clearly observed a reduction in the total serum levels of IL-6 in TDP-43-depleted mice ( Fig. 8e ). However, levels of IL-10 in the serum of mice were barely detected at the indicated times, because IL-10 is mainly secreted at later time points during LPS stimulation. Consistent with in vitro data from primary cells, these results strongly indicate that TDP-43-mediated InSACs induce LPS-mediated inflammation by facilitating IL-6 RNA processing. 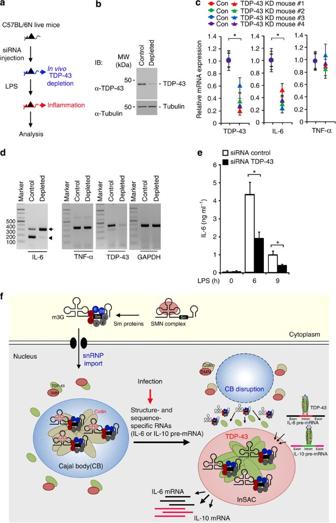Figure 8: TDP-43 is essential for IL-6 RNA processing. (a–e)In vivoTDP-43 depletion impairs IL-6 production. (a) Strategy for depletion of TDP-43in vivoand development of inflammation by LPS. C57BL/6N mice were divided into two different groups, namely control mice injected with the control-Invivofectamine complex (n=4) and an experimental group injected with the TDP-43 siRNA-Invivofectamine complex (n=4). Each siRNA-Invivofectamine complex was intraperitoneally administered and then the mice were treated intraperitoneally with LPS (5 mg kg−1) to induce inflammation. Serum was collected at 0, 6 and 9 h for ELISA. After 9 h, mice were euthanized and the splenic macrophages were collected for RT–PCR, qRT–PCR or immunoblot analysis. (b) The efficiency of TDP-43 depletion in splenic macrophages was confirmed by immunoblot analysis using anti-TDP-43 or anti-β-actin antibody. (c) qRT–PCR with Taqman showed a significant reduction in IL-6 mRNA production. All qRT–PCR data were normalized to the expression of GAPDH mRNA. (n=4), *P<0.005 (Student’st-test). (d) RT–PCR using primer pairs (P1) for the exon 1–exon 2 junction of IL-6 RNA was performed from control or TDP-43-depleted mice. Confirmation of TDP-43 knockdown and measurement of the quantity of RNA were achieved by RT–PCR with primer pairs P4, P6 and P7. Arrowheads and arrows indicate mRNA and pre-mRNA, respectively. (e) ELISA assay was carried out to measure IL-6 levels in serum from control or TDP-43-depleted mice. (n=4), *P<0.01 (Student’st-test). (f) Model of TDP-43-mediated subnuclear foci function in IL-6 and IL-10 pre-mRNA processing. Data are representative of at least three independent experiments (mean±s.e.m. inc; mean±s.d. ine). Figure 8: TDP-43 is essential for IL-6 RNA processing. ( a – e ) In vivo TDP-43 depletion impairs IL-6 production. ( a ) Strategy for depletion of TDP-43 in vivo and development of inflammation by LPS. C57BL/6N mice were divided into two different groups, namely control mice injected with the control-Invivofectamine complex ( n =4) and an experimental group injected with the TDP-43 siRNA-Invivofectamine complex ( n =4). Each siRNA-Invivofectamine complex was intraperitoneally administered and then the mice were treated intraperitoneally with LPS (5 mg kg −1 ) to induce inflammation. Serum was collected at 0, 6 and 9 h for ELISA. After 9 h, mice were euthanized and the splenic macrophages were collected for RT–PCR, qRT–PCR or immunoblot analysis. ( b ) The efficiency of TDP-43 depletion in splenic macrophages was confirmed by immunoblot analysis using anti-TDP-43 or anti-β-actin antibody. ( c ) qRT–PCR with Taqman showed a significant reduction in IL-6 mRNA production. All qRT–PCR data were normalized to the expression of GAPDH mRNA. ( n =4), * P <0.005 (Student’s t -test). ( d ) RT–PCR using primer pairs (P1) for the exon 1–exon 2 junction of IL-6 RNA was performed from control or TDP-43-depleted mice. Confirmation of TDP-43 knockdown and measurement of the quantity of RNA were achieved by RT–PCR with primer pairs P4, P6 and P7. Arrowheads and arrows indicate mRNA and pre-mRNA, respectively. ( e ) ELISA assay was carried out to measure IL-6 levels in serum from control or TDP-43-depleted mice. ( n =4), * P <0.01 (Student’s t -test). ( f ) Model of TDP-43-mediated subnuclear foci function in IL-6 and IL-10 pre-mRNA processing. Data are representative of at least three independent experiments (mean±s.e.m. in c ; mean±s.d. in e ). Full size image These studies identify and characterize the InSAC as a novel subnuclear site enriched with TDP-43, IL-6 and IL-10 cytokine pre-mRNAs, snRNAs and Sm proteins. InSAC bodies form in a cell type capable of producing TDP-43-binding cytokine RNAs. Our study also elucidates how IL-6 and IL-10 pre-mRNA processing is tightly regulated by TDP-43-mediated InSAC formation, and how this regulation may be maintained during the immune response to microbial infection. TDP-43 functions as a scaffolding protein that is required for competitively recruiting critical spliceosomal components, thereby facilitating specific cytokine pre-mRNA processing and preventing its degradation. The RNA-binding selectivity of TDP-43 is determined by sequence-specific recognition, leading to the induction of IL-6 and IL-10 RNA processing. In addition, TDP-43-targeted RNA contains GC-rich palindromic repeats along with the conserved ‘ACU’ sequence motifs within a short spacer region. Ultimately, TDP-43-mediated InSAC formation is important in promoting immune defense mechanisms against microbes and maintaining immune homeostasis ( Fig. 8f ). In particular, ‘ACU’ sequence motifs within the short spacer region of human IL-6 intron 1 are similar to that of mouse IL-6 intron 2 and mouse IL-10 intron 1. In addition, compared with mouse IL-10, human IL-10 intron 2 also contained the conserved GC-rich palindromic sequences and ‘ACC’ instead of ‘ACU’ within a short spacer region ( Supplementary Fig. 4 ). Thus, it remains possible that TDP-43 may contribute to the enhancement of human IL-6 and IL-10 RNA processing. In contrast, TDP-43 does not influence RNA splicing of TNF-α, IL-12, IL-8 or IL-1β, the major proinflammatory cytokines elicited by LPS or CpG-DNA stimulation. We have been unable to identify a predicted stem-loop sequence within their introns. Although some contain GC-rich palindromic repeats, they possess a larger spacer instead of a short spacer consisting of five or six nucleotides. Presumably, a putative large stem-loop within an intron is unfavourable for the TDP-43 interaction ( Figs 3c and 4a , and Supplementary Fig. 3 ). This raises the question of whether additional specialized nuclear compartments exist that interact with cytokine RNAs containing uncharacterized structural elements, such as a large stem-loop or helix, leading to the selective processing of these cytokine RNAs. TDP-43 plays an important role in competitively nucleating essential spliceosomal components to InSACs from CBs in response to LPS, and in controlling the distribution of subnuclear compartments as well ( Fig. 5 ). Previous studies have shown that coilin is a multivalent scaffold, allowing it to bind snRNPs efficiently through low-affinity interactions with CB components including SMN [32] , [33] , [34] , and that subnuclear snRNAs are specifically required for CB formation [35] , [36] .Thus, it seems likely to be that the LPS-induced high-affinity interaction of coilin with SMN prevents the binding of coilin to snRNAs, thereby destabilizing CB formation; on the other hand, the LPS-mediated low-affinity interaction of TDP-43 with SMN may enhance the association of TDP-43 with snRNAs, thus stabilizing InSACs. TLRs recognize different components from bacteria, fungi and viruses to produce various cytokines and chemokines that are critical for inducing innate and adaptive immune responses [27] . As TLR4 is essential for LPS recognition, many adaptor proteins involved in activating this receptor could also be critical in LPS-induced TDP-43 modifications. Previous studies have shown that TDP-43 function is affected by a deficiency in progranulin [37] , a secreted protein that regulates multiple pathways involved in nucleic acid-sensing TLR9 activation [38] , [39] . However, a correlation between TDP-43 and progranulin in LPS-induced InSAC formation remains unclear and might be a subject for future investigation. In particular, Swarup et al . [25] has shown that physical interaction between TDP-43 and NF-κB p65 promotes NF-κB-mediated neuroinflammation in ALS cases and TDP-43 transgenic mice. Importantly, we show that InSAC formation is normal in N2A cells even without LPS stimulation. Moreover, the expression of the IL-6 minigene was efficiently processed to mature RNA in the absence of LPS stimulation. Therefore, regardless of NF-κB activation, InSAC formation seems to occur through the recruitment and accumulation of spliceosomal components by recruiting sequence- and structure-specific RNAs, but the possibility remains of the involvement of NF-κB in regulating InSAC formation or the dynamic distribution of other subnuclear bodies. IL-6 is a pleiotropic cytokine that functions broadly in immune and non-immune cells as a pro- and anti-inflammatory cytokine [11] . A very recent publication by Shalek et al . [40] has reported that IL-6 is a sustained cytokine, which continues to show high expression over 12 h after LPS stimulation, compared with TNF-α, which is produced for a very short time during infection. We noted that the InSAC appears at 1 h after LPS stimulation and increases in size in a time-dependent manner. It is possible that InSAC size may be highly correlated with IL-6 RNA production. We thus assume that autoimmune diseases or cancers could be characterized by excessive InSAC formation, and that these conditions could arise due to abnormal TDP-43 modifications, such as ubiquitination or oligomerization. Such insights into the molecular pathology of various cancers and autoimmune diseases may accelerate the development of improved therapies for treating these diseases. DNA constructs Mouse TDP-43 constructs were fused at the N terminus to haemagglutinin (HA) or GFP, and mouse Coilin was tagged at the C terminus with Myc. All constructs were cloned into the retroviral pMSCV (puro) or pLHCX (hygro) vector (Clontech, Mountain View, CA). The shRNA sequence against TDP-43, GFP and UBE2E3 was annealed and subcloned into the pSUPER retroviral vector (Oligoengine, Seattle, WA). Myc-IL-6 minigene comprising exon 1, intron 1, exon 2, intron 2 and exon 3 was constructed by PCR amplification from genomic DNA and subcloned in pMSCV N-term Myc, between the XhoI and EcoRI sites. The mutant minigene of IL-6 was generated by overlap extension PCR. All constructs were verified by sequencing and all primer sequences are listed in Supplementary Table 2 . Antibodies Antibodies against Myc (1:2,000; 2276), HA (1:1,000; clone 3F10 and 12CA5) and GFP (1:4,000; ab290) were obtained from Cell Signaling Technology (Danvers, MA), Roche (Basel, Switzerland) and Abcam (Cambridge, UK), respectively. The following antibodies were also used: anti-TDP-43 (1:500; A303-223A; Bethyl Laboratories, Montgomery, TX, and 1:1,000 ab104223; Abcam), anti-Coilin (1:200; sc-32860 and sc-135871; Santa Cruz Biotechnology, Santa Cruz, CA), anti-Promyelocytic Leukemia (1:200; AM20293AF-N; Acris Antibodies, San Diego, CA), anti-Nucleolin (1:200; sc-55486; Santa Cruz), anti-SMN (1:2,000; 610646; BD Biosciences, San Jose, CA), anti-Sm (1:1,000; MS-450-P; Thermo Scientific, Fremont, CA), anti-2,2,7-Trimethylguanosine (1:500; NA02; Merck KGaA, Darmstadt, Germany) and anti-UBE2E3 (1:1,000; Merck Millipore, clone MABS17). Antibodies against ubiquitin (1:1,000; 13-160), phospho-serine (1:200; 61-8100) and SUMO-1 (1:2,000; S8070) were purchased from Life Technologies (Carlsbad, CA) and Sigma (St Louis, MO). Mice and cell lines C57BL/6 mice were purchased from the Jackson Laboratory. All mice were maintained in the specific pathogen-free facility of the Yonsei Laboratory Animal Research Center at Yonsei University. Murine RAW264.7 macrophages (TIB71, ATCC, Manassas, VA) human embryonic kidney 293T cells (CRL-3216, ATCC) and NF-κβ p65-deficient MEFs (kindly provided by Dr Alxander Hoffmann) were cultured in DMEM supplemented with 10% heat-inactivated fetal bovine serum (HyClone, Logan, UT) and penicillin/streptomycin (HyClone). Cells were grown at 37 °C in humidified air with 5% CO 2 . Generation of BMDCs and BMDMs BMDMs and BMDCs were generated from wild-type C57BL/6 mice (Orient Bio, Gyeonggi-do, South Korea), in medium containing macrophage colony-stimulating factor (CSF) (BioLegend, San Diego, CA) or granulocyte macrophage-CSF (BioLegend). Briefly, femurs and tibiae were collected from mice 4–5 weeks old. After removing bone adjacent muscles, marrow cells were extracted by flushing with a 25-gauge needle. Bone marrow cells were then resuspended on DMEM medium (10% fetal bovineserum and 1% antibiotics) with macrophage-CSF (25 ng ml −1 ) or granulocyte macrophage-CSF (5 ng ml −1 ). Fresh medium was replenished on days 2 and 4. BMDMs and BMDCs were generated after 6–8 days of culture. Retroviral transduction Human embryonic kidney 293T cells were transfected with plasmids encoding VSV-G and Gag-Pol, as well as either coilin-Myc, HA-TDP-43, GFP-TDP-43, negative control shRNA for GFP, shRNA for TDP-43, or shRNA for UBE2E3. Thirty-six to 48 h post transfection, media containing viral particles were collected, filtered through a 0.45-μm membrane and incubated with RAW macrophages for 24 h. Cells were selected with puromycin or hygromycin. Enzyme-linked immunosorbent assay RAW264.7 macrophages expressing control shRNA against GFP or shRNA against TDP-43 or UBE2E3 were cultured with LPS (80 ng ml −1 ) for 6 h. BMDMs or BMDCs was transfected (DharmaFECT, Thermo Scientific) with either scrambled siRNA or TDP-43 siRNA for 48 h, followed by stimulation with LPS (80 ng ml −1 ) or CpG-DNA (1 μM) for 6 h. Tissue culture supernatants were collected, and mouse IL-6, IL-10 and TNF-α levels were analysed by ELISA assay according to the manufacturer’s recommendations (BD Biosciences). RNA immunoprecipitation Nuclear fractions were isolated using a hypotonic buffer containing 10 mM HEPES, pH 7.9, 15 mM MgCl 2 , 10 mM KCl, 0.05% NP-40 and protease inhibitor cocktail (Roche). Nuclear extracts were resuspended in RIP buffer (50 mM Tris-Cl, pH 7.4, 300 mM NaCl, 0.05% NP-40 and protease inhibitor cocktail) containing 100 units of RNase inhibitor (TaKaRa, Otsu, Japan) and then incubated with anti-HA or anti-Isotype control antibody overnight. After incubation with protein G-Sepharose beads (Sigma) for 1 h, samples were washed with ice-cold RIP buffer and RNA was extracted using an RNA purification kit (GeneAll, Seoul, South Korea) according to the manufacturer’s instructions. All primer sequences are listed in Supplementary Table 1 . GST pull-down and RNA electrophoretic mobility shift assay Escherichia coli -expressed GST-TDP-43 was purified by Glutathione-agarose (Sigma) according to the supplier’s instructions, with minor modifications. The binding reaction was performed by mixing the purified GST-TDP-43 with biotin-labelled RNA for IL-6 intron 2 (biotin-5′- AUGCCUCCCAGC AC UU GGGAGG CAC -3′) or mutated RNAs; mutCA+GUUUCUU (biotin-5′- AUGCCUCCCAGC CA U GUUUCUU CAC -3′), mutGU (biotin-5′- AUGCCUCCCAGC GU UUGGGAGGCAC -3′), or mutUUU (biotin-5′- AUGCCUCCCAGCACUU UUU AGGCAC -3′) in 20 μl reaction buffer according to the manufacturer’s protocol (LightShift Cmiluminescent RNA EMSA Kit, Thermo Scientific, Rockford, IL). Reaction mixtures were separated by a 6% native acrylamide gel in 0.5 × TBE and further analysed by streptavidin–horseradish peroxidase (Thermo scientific). In vivo RNA interference experiment TDP43 expression in live mice was knocked down by siRNA to TDP43 with Invivofectamine (Invitrogen). siRNA–Invivofectamine complex was prepared as per the manufacturer’s protocol. Briefly, siRNAs (3 mg ml −1 ) were mixed with complexation buffer and Invivofectamine, incubated for 30 min at 50 °C and dialysed at room temperature for 2 h in PBS (pH 7.4). Dialysed siRNA-Invivofectamine complex (7 mg kg −1 ) was intraperitoneally injected through female C57BL/6 (5 or 6 weeks) mice. Two days later, mice were treated intraperitoneally with LPS (5 mg kg −1 ). After 9 h, mice were euthanized and the spleens were collected for RT–PCR or qRT–PCR. To purify splenic macrophages, the spleens were dissected from abdominal cavity and removed red cells. Flow cytometry sorting was performed to obtain F4/80-positive and CD11c-negative cells. Mouse serum was collected at 0, 6 and 9 h for ELISA assay. Real time PCR Total cellular RNA was prepared using an RNA prep kit (GeneAll). Next, 500 ng total RNA was reverse transcribed for 1 h with random hexamers at 42 °C using M-MLV (Moloney Murine Leukemia Virus) reverse transcriptase (Enzynomics, Seoul, South Korea). Subsequently, PCR was performed using the following conditions: 30 cycles of 15 s at 94 °C, 15 s at the experimentally determined optimal annealing temperature (at 56–58 °C) and 60 s per 1 kb at 72 °C (15–40 s). PCR products were visualized on ethidium bromide-stained gels. Glyceraldehyde 3-phosphate dehydrogenase (GAPDH) was used for normalization. Real-time PCR was performed using TOPreal qPCR premix (SYBR Green, Enzynomics) and Applied Biosystems 7300 Real-Time PCR System (Life Technologies). TaqMan quantitative PCRs were performed with TaqMan gene expression assays (Applied Biosystems) for TDP-43 (Mm00523866_m), IL-6 (Mm00446190_m1), TNF-α (Mm00443258_m1) and GAPDH (Mm99999915_g1). Results were normalized to expression of the gene encoding GAPDH and were quantified by the change-in-threshold method (ΔΔCT). All primer sequences and the predicted band sizes are listed in Supplementary Table 1 . Immunofluorescence assay For immunofluorescent staining, cells were fixed in 3.7% formaldehyde and permeabilized with 0.1% Triton X-100 before incubation with the appropriate primary antibody. Bound antibody was visualized with an Alexa Fluor 488- or Alexa Fluor 568-conjugated secondary antibody (Life Technologies). DAPI (4′, 6-diamidino-2-phenylindole) (Sigma) was used as a nuclear counterstain. FISH assay Cells were fixed with 3.7% formaldehyde and permeabilized with 70% Ethanol. Cy3-labelled probes for IL-6 intron 2 (Cy3-5′- AGCATAGAGTAGGAACTTGGTAAAGGACAG -3′) was incubated with hybridization buffer (10% formamide, 2 × SSC, Dextran sulfate (100 mg ml −1 )) and RNase inhibitor (100 unit) at 37 °C for 4 h in a humid dark box. Unbound probe was removed by washing buffer (10% formamide and 2 × SSC). Immunoprecipitation and immunoblot analysis Approximately 2.5 × 10 6 cells were lysed with 2% NP-40 in PBS supplemented with protease inhibitors for 1 h at 4 °C. Lysates were first precleared with protein G-Sepharose beads (Sigma) before the addition of primary antibodies followed by protein G-Sepharose beads. The samples were incubated at 4 °C. The beads were then washed five times with 0.2% NP-40/PBS and proteins were eluted by boiling the samples in denaturing buffer. Proteins were separated by SDS–PAGE, transferred onto a nitrocellulose membrane, blocked with 5% skim milk in PBS containing 0.1% Tween-20 (Sigma) for 2 h and then probed with the appropriate antibody for 4 h at room temperature. Membranes were washed three times with PBS containing 0.1% Tween-20 and incubated with horseradish peroxidase-conjugated streptavidin for 1 h. Bands were visualized using an ECL detection reagent (Thermo Scientific). Ethics statement All animal experiments were performed in accordance with the Korean Food and Drug Administration guidelines. Protocols were reviewed and approved by the Institutional Animal Care and Use Committee of the Yonsei Laboratory Animal Research Center at Yonsei University (Permit Number: 2007-0001). Statistical analysis All experiments were repeated at least three times with consistent results. Data are presented as mean and s.d. or s.e.m (as noted in figure legends). Statistical differences between two means were evaluated with the two-tailed unpaired Student’s t -test. Differences with P -values below 0.05 were considered significant. No samples were excluded from the analysis. The data had a normal distribution and the variance was similar between the groups being statistically compared. No statistical method was used to predetermine sample sizes. Sample size was based on previous experience with experimental variability. The experiments were not randomized. The investigators were not blinded to allocation during experiments or outcome assessment. How to cite this article: Lee, S. et al . Identification of a subnuclear body involved in sequence-specific cytokine RNA processing. Nat. Commun. 6:5791 doi: 10.1038/ncomms6791 (2015).